Wafer-scale design of lightweight and transparent electronics that wraps around hairs Electronics on very thin substrates have shown remarkable bendability, conformability and lightness, which are important attributes for biological tissues sensing, wearable or implantable devices. Here we propose a wafer-scale process scheme to realize ultra flexible, lightweight and transparent electronics on top of a 1-μm thick parylene film that is released from the carrier substrate after the dissolution in water of a polyvinyl– alcohol layer. The thin substrate ensures extreme flexibility, which is demonstrated by transistors that continue to work when wrapped around human hairs. In parallel, the use of amorphous oxide semiconductor and high-K dielectric enables the realization of analogue amplifiers operating at 12 V and above 1 MHz. Electronics can be transferred on any object, surface and on biological tissues like human skin and plant leaves. We foresee a potential application as smart contact lenses, covered with light, transparent and flexible devices, which could serve to monitor intraocular pressure for glaucoma disease. Flexible electronic circuits are essential for the development of fully flexible systems, which would enable new applications in electronics, biotechnology, energy and sensing [1] , [2] , [3] , [4] . Rollable displays [5] , [6] , [7] , conformable sensors [8] , plastic solar cells [9] , [10] and flexible batteries [9] , [10] , [11] promise to change our daily life like CMOS technology did in the past decades. So far, the effective commercialization of such technologies has been mainly prevented by cost and performance constraints. However, for some applications, like medical or implantable devices, the specific functionalities provided by flexible, biocompatible, conformable and light plastic electronics are much more important than the aforementioned obstacles and future scenarios can be realistically foreseen. The development of flexible electronic circuits plays a crucial role in all such applications [12] , [13] , [14] , [15] . Flexibility in thin film devices can be achieved by direct fabrication on plastic foil [16] , by peeling off a polymer layer spin coated on a rigid substrate [17] or by spalling the thin top layer from a crystalline silicon wafer after device fabrication [18] . Extremely small bending radii (<1 mm) can be achieved either by using materials with high mechanical strength [19] , [20] , [21] or by fabricating the electronics in the neutral strain position [22] . In addition to the two aforementioned strategies, a third very promising route consists in the use of ultrathin substrates [19] , [23] , [24] , [25] , [26] . Besides the extreme bendability, this approach offers unique capabilities as lightness and conformability, which are important for smart-skin [24] , [27] , biological tissue sensing [28] and even solar cells [25] . The substrate can be also chosen to accomplish specific functions like dissolution after a predetermined time frame [29] . In this study, we propose a method to achieve ultra flexible electronics on an engineered substrate, which is not only a useful support during the fabrication, but whose thickness and properties are designed according to the desired application. We realize electronics on top of a bi-layer polymer substrate, which can be selectively dissolved to enable the release from a hosting support, the transfer and the adhesion onto almost any surface and the removal after use. Following this approach, sensors, transistors and circuits have been micro machined on top of a 1-μm thick parylene film, which is released from a carrier chip after the dissolution of a PVA layer in water. Transparent and non-transparent transistors based on amorphous-indium gallium zinc oxide (a-IGZO) have mobility as high as 16 cm 2 V −1 s −1 and 24 cm 2 V −1 s −1 , respectively, and continue to work even when wrapped around hairs with a radius of 50 μm. Transparent and lightweight devices are transferred on plastic contact lenses, which could potentially be used to monitor the intraocular pressure for glaucoma. The possibility to implement such scheme at wafer scale and the use of a-IGZO could represent a good compromise between large area integration and performance and, hence, a valid alternative to similar reported approaches [24] , [27] (see Supplementary Table S1 for a comparison with literature data). 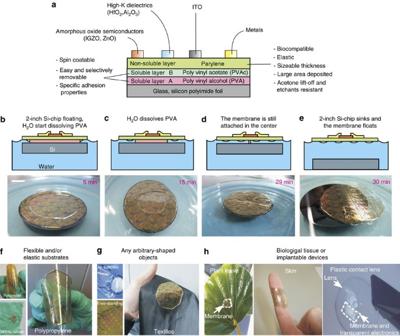Figure 1: Materials, process and methodology to realize ultra flexible electronics. (a) The proposed engineered substrate consists of two soluble films (PVA and PVAc) and of a non-soluble layer (parylene) deposited on rigid or flexible support. The selective dissolution of the layers enables the release, the transfer, the adhesion and the removal after use of the electronics. The desired requirements for the layers are listed in bold. Low-temperature processable materials can be employed to fabricate ultra flexible devices in electronics and photonics. (b–e) The proposed process scheme can be implemented at wafer scale. Here, we demonstrate the feasibility of such approach in the case of a 2-inch wafer. The water starts dissolving the PVA layer from the borders of the wafer and slowly proceeds towards the centre. The whole releasing procedure takes ~30 min after which the wafer sinks while the membrane floats on water (Scale bar in b, 1 cm). (f–h) After the release of the hosting support, the membrane is fished and transferred onto flexible and elastic foils, textiles, biological tissues and implantable devices. In case of transfer to polyimide foils, nitride rubber, plant leaves and human skin, we dissolved an additional PVAc film in acetic acid to remove the electronics after use. Concept Figure 1a illustrates the idea behind our work. Two or more polymer films can be deposited by spin coating on a rigid or flexible support. Each of them is easily and selectively removable by a specific solvent, while some could have specific properties like good adhesion. On top of the stack lays a non-soluble layer, which constitutes the ultimate substrate film and which is released from the support after the dissolution of soluble layers. Depending on the applications, it can be chosen to be biocompatible, elastic and its thickness tuned to set the desired final flexibility. It must be resistant to the solvents, which dissolve the underlying stack and possibly to solvents and etchants used for the structuring of the active electronic layers. In Fig. 1a , we listed some of the materials that could fulfil such requirements. Regarding the active layers that form the electronic components, low-temperature (<150 °C) processable materials are compatible with our process scheme. This could include a complete set of basic electronic ingredients, that is, semiconductors (amorphous oxide semiconductors), metals and high-K dielectrics. A similar approach has been used to realize flexible molybdenum disulphide, MoS 2 , transistors [30] . Such large spectrum of possibilities can lead to ultra flexible devices in electronics and photonics and find application in ultralight solar cells, implantable devices, rollable and transparent displays, smart-skin and electronic textiles. Figure 1: Materials, process and methodology to realize ultra flexible electronics. ( a ) The proposed engineered substrate consists of two soluble films (PVA and PVAc) and of a non-soluble layer (parylene) deposited on rigid or flexible support. The selective dissolution of the layers enables the release, the transfer, the adhesion and the removal after use of the electronics. The desired requirements for the layers are listed in bold. Low-temperature processable materials can be employed to fabricate ultra flexible devices in electronics and photonics. ( b – e ) The proposed process scheme can be implemented at wafer scale. Here, we demonstrate the feasibility of such approach in the case of a 2-inch wafer. The water starts dissolving the PVA layer from the borders of the wafer and slowly proceeds towards the centre. The whole releasing procedure takes ~30 min after which the wafer sinks while the membrane floats on water (Scale bar in b, 1 cm). ( f – h ) After the release of the hosting support, the membrane is fished and transferred onto flexible and elastic foils, textiles, biological tissues and implantable devices. In case of transfer to polyimide foils, nitride rubber, plant leaves and human skin, we dissolved an additional PVAc film in acetic acid to remove the electronics after use. Full size image Non-transparent electronics on 1 μm parylene film To demonstrate the feasibility of this approach we micro machined passive components, thin film transistors (TFTs) and circuits on top of a 1-μm thick parylene film. Parylene is chosen because it is biocompatible [31] , [32] and resistant to acetone and chemicals necessary for lift-off and etching process steps (see Methods and Supplementary Fig. S1 ). In our experiments, PVA constitutes the first soluble layer needed to release, in water, the silicon wafer used as support during the fabrication ( Fig. 1b–e ). Depending on the application, an additional polyvinyl acetate (PVAc) film is added to improve the adhesion and enable the removal of electronics after use. The PVA and PVAc layers have a thickness of about 400 nm and are spin coated, while parylene is thermally evaporated. Following the substrate preparation, TFTs were fabricated. The semiconductor is a 15 nm thick layer of sputtered a-IGZO while the gate dielectric consists of 25-nm thick Al 2 O 3 deposited by atomic layer deposition. Source and drain contacts are formed by 10 nm/60 nm of evaporated Ti/Au layers. A 25 nm thin film of Al 2 O 3 is used to passivate the structures and improve the environmental stability of the devices. The maximum process temperature is 150 °C reached during the atomic layer deposition dielectric deposition. The final thickness of the TFT structure is 145 nm (see Supplementary Fig. S2 for the device layout and structure). In order to test and prove the reliability of our approach, we also designed and fabricated analogue amplifiers based on the previously described TFTs. It is worth mentioning that the use of rigid supports (glass or silicon) during the fabrication, mitigate some issues, like substrate thermal expansion or water absorption, which are encountered in case of direct fabrication on foils and which limit the feature resolution and alignment, therefore, yield and performance. After the fabrication, the chip was put in water to selectively dissolve the PVA layer and release the parylene membrane. For a 2-inch wafer, this operation takes ~30 min after which the circuits are floating on water ( Fig. 1b–e ). The membrane can then be fished and transferred onto the final destination substrate, which can be any arbitrary rigid or flexible support or any organic or inorganic surface (see Fig. 1f–h and Supplementary Fig. S6 ). As first demonstration, we transferred it onto a 50-μm thick polyimide foil that we dipped into the water, moved beneath the membrane and then lifted up. The membrane and the foil were baked for 10 min at 70 °C to evaporate the remaining water and to improve the adhesion. A flexible foil with the transferred electronics is shown in Supplementary Fig. S2 while devices before and after transfer are shown in Fig. 2a,b , respectively. It is worth mentioning that no wrinkles or cracks are observed after the process. 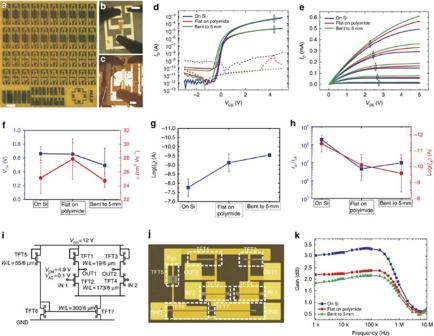Figure 2: TFTs and circuits transferred on a flexible polyimide foil. (a) Bottom gate transistors fabricated on a parylene/PVAc/PVA/silicon template (ground signal ground, GSG, layout) (scale bar, 500 μm). (b) Device after transfer onto a 50-μm thick polyimide foil. The adhesion between parylene and Kapton is good after baking at 70 °C for 10 min. No wrinkles or cracks are visible (scale bar, 100 μm). (c) Device bent down to 5 mm (ε=0.5%) (scale bar, 100 μm). (d) Transfer characteristic (VDS=0.1, 5 V) of a typical a-IGZO TFT (channel width/length of 50 μm per 9 μm). The device is measured on Si, transferred onto the foil and then bent to a tensile radius of 5 mm parallel to the TFT channel (dotted lines in theIDS-VGScurve represent the gate leakage current). (e) Output (VGS=1, 2, 3, 4, 5 V) characteristic of the device shown ind. (f–h) After the transfer, 17 devices work out of 20 measured on Si (yield of 85%) and all devices continue to work when bent. Threshold voltage,VTH, remains almost constant while the mobility,μ, shows an average value of 26 cm2V−1s−1with an increase when transferred onto polyimide and then a decrease during bending test. Gate leakage,IG, decreases by more than a decade on polyimide and remains smaller than 1 nA during bending (plot in logarithmic scale). Off-state current,Ioff, (plot in logarithmic scale), instead, increases and, consequently, theIon/Ioffratio decreases while remaining always greater than 106. In addition, an average decrease of the output resistance by 50% and a slight deterioration of the sub-threshold swing are also observed. Errors bars in the plots indicate the s.d. (i) Schematic of a differential amplifier constituted by 7 TFTs, which have a channel length as small as 6 μm. The output signals are measured by two active probes (C⩽2 pF,R=1 MΩ). The supply voltage (VDD) is 12 V. (j) Photograph of the differential amplifier after fabrication. (k) The bode plot of the amplifier shows a bandwidth of about 1 MHz and the gain is about 3, 2.2 and 1.7 dB, respectively on silicon, on polyimide and under bending. The gain degradation could be due to the TFTs threshold voltage shift and the decrease of the output resistance observed after the transfer. Figure 2: TFTs and circuits transferred on a flexible polyimide foil. ( a ) Bottom gate transistors fabricated on a parylene/PVAc/PVA/silicon template (ground signal ground, GSG, layout) (scale bar, 500 μm). ( b ) Device after transfer onto a 50-μm thick polyimide foil. The adhesion between parylene and Kapton is good after baking at 70 °C for 10 min. No wrinkles or cracks are visible (scale bar, 100 μm). ( c ) Device bent down to 5 mm ( ε =0.5%) (scale bar, 100 μm). ( d ) Transfer characteristic ( V DS =0.1, 5 V) of a typical a-IGZO TFT (channel width/length of 50 μm per 9 μm). The device is measured on Si, transferred onto the foil and then bent to a tensile radius of 5 mm parallel to the TFT channel (dotted lines in the I DS - V GS curve represent the gate leakage current). ( e ) Output ( V GS =1, 2, 3, 4, 5 V) characteristic of the device shown in d . ( f – h ) After the transfer, 17 devices work out of 20 measured on Si (yield of 85%) and all devices continue to work when bent. Threshold voltage, V TH , remains almost constant while the mobility, μ , shows an average value of 26 cm 2 V −1 s −1 with an increase when transferred onto polyimide and then a decrease during bending test. Gate leakage, I G , decreases by more than a decade on polyimide and remains smaller than 1 nA during bending (plot in logarithmic scale). Off-state current, I off , (plot in logarithmic scale), instead, increases and, consequently, the I on / I off ratio decreases while remaining always greater than 10 6 . In addition, an average decrease of the output resistance by 50% and a slight deterioration of the sub-threshold swing are also observed. Errors bars in the plots indicate the s.d. ( i ) Schematic of a differential amplifier constituted by 7 TFTs, which have a channel length as small as 6 μm. The output signals are measured by two active probes ( C ⩽ 2 pF, R =1 MΩ). The supply voltage ( V DD ) is 12 V. ( j ) Photograph of the differential amplifier after fabrication. ( k ) The bode plot of the amplifier shows a bandwidth of about 1 MHz and the gain is about 3, 2.2 and 1.7 dB, respectively on silicon, on polyimide and under bending. The gain degradation could be due to the TFTs threshold voltage shift and the decrease of the output resistance observed after the transfer. Full size image The transistors and circuits were electrically characterized before ( Fig. 2a ) and after the transfer ( Fig. 2b ) and bent down to 5 mm radii ( Fig. 2c ), which corresponds to 0.5% strain [33] level parallel to the TFT channel. A typical device, measured on the silicon carrier (blue curve in Fig. 2d,e ), exhibits a field effect mobility of 23 cm 2 V −1 s −1 and a threshold voltage of 0.36 V. The off-current (drain current at V GS =0 V) is as low as 50 fA μm −1 with an I on / I off >10 7 . After the transfer, the same devices (red curve in Fig. 2d,e ) show a smaller gate leakage current, a slight shift of the threshold voltage and a deterioration of the output resistance. The Al 2 O 3 passivation film ensures good environmental stability preventing any water absorption [34] , which is experimentally proved by hysteresis-free I D − V GS curves. The green curves in Fig. 2d,e demonstrate that the TFTs stay fully functional when bent to 5 mm. They exhibit a slightly increased I on , as expected from IGZO TFTs under tensile strain [35] . Our previous studies demonstrate that similar devices on a 50-μm thick polyimide foil cannot stand strain level greater than 0.5% due to the formation of cracks in the gate stack [14] . The transfer process is reproducible and robust (yield of 85%) and repeated measurements on several devices ( Fig. 2f–h ) show an almost constant threshold voltage, gate leakage, which is always smaller than 1 nA and I on / I off greater than 10 6 . These findings encouraged the realization of circuits. Figure 2i,j shows, respectively, the schematic and a photograph after fabrication of a differential amplifier, which operates at 12 V and composed by seven TFTs. When measured on silicon, it has a bandwidth of about 1 MHz and a gain of 3 dB (blue curve in Fig. 2k ), which decreases to 2 dB after bending to 5 mm (green curve in Fig. 2k ) due to the reduced output resistance observed in the TFTs. The bandwidth remains unaltered. Such circuit can be potentially used for signal amplification in smart skin application. Transparent TFTs In order to take advantage of the transparency of the parylene membrane and of a-IGZO, fully transparent TFTs were fabricated by replacing the gate and source/drain metal contacts with 100 nm ITO film, which is sputtered at room temperature (see Supplementary Fig. S3 ). The transparent devices were also transferred on a polyimide foil and their electrical response to applied strain was studied as in case of Ti/Au TFTs. It is worth mentioning that after the transfer, some wrinkles appear in the ITO films ( Fig. 3b–d ) while they were not present in case of non-transparent devices ( Fig. 2b and Supplementary Fig. S2c ). Such wrinkles are due to built-in strain in the ITO layer. Despite the fact that they do not prevent the devices to work properly ( Fig. 3e,f ), a higher gate leakage current ( Fig. 3i ) is observed after the transfer and a lower yield is registered if compared with non-transparent electronics (the latter point, at the moment, prevent the realization of transparent circuits). Measurements shown in Fig. 3e (transfer characteristic) and Fig. 3f (output characteristic) demonstrate that ITO transistors continue to work when bent down to 10 mm ( ε =0.25%) and 6 mm ( ε =0.4%) with no hysteretic behaviour. They exhibit an average mobility of 16 cm 2 V −1 s −1 , a threshold voltage of 0.2 V ( Fig. 3g ) and an I on / I off ratio, which remains greater than 10 4 ( Fig. 3h ). Higher strain levels provoke cracks and delamination of the ITO layer, which irreversibly hamper the proper operation of the devices. 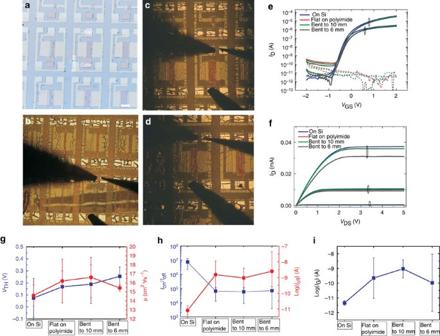Figure 3: Transparent TFTs transferred on polyimide foil. (a) Transparent TFTs have been fabricated by replacing metals with transparent ITO (Scale bar, 100 μm). (b) The devices are transferred on a polyimide foil. After the transfer wrinkles are observed in the ITO layer. The wrinkles were not present in the case of Ti/Au metallization (Fig. 2b) and they are due to built-in stress in the ITO film. (c) Devices bent to 10 mm (ε=0.25%). (d) Devices bent to 6 mm (ε=0.4%). (e) Transfer characteristic (VDS=0.1, 5 V) of aW/L=280 μm/60 μm transparent TFT, which is measured on Si, flat on polyimide after transfer and then bent to 10 and 6 mm (tensile strain parallel to the channel). Higher strain levels provoke cracks and delamination of the ITO. (f) Output characteristics forVGS=1, 1.5, 2 V of the device shown ine. (g–i) The transfer yield is about 50% (10 devices out of 20 work after transfer). The most remarkable changes, after the transfer, are observed in the increase of the gate leakage,IG, ((i) plot in logarithmic scale) and of the off-current,Ioff, ((h) plot in logarithmic scale). Threshold voltage,VTH, remains, instead, stable and average mobility,μ, is of about 16 cm2V−1s−1, which is lower than the Ti/Au metallization because of the increased contact resistance. Errors bars in the plots indicate the s.d. Figure 3: Transparent TFTs transferred on polyimide foil. ( a ) Transparent TFTs have been fabricated by replacing metals with transparent ITO (Scale bar, 100 μm). ( b ) The devices are transferred on a polyimide foil. After the transfer wrinkles are observed in the ITO layer. The wrinkles were not present in the case of Ti/Au metallization ( Fig. 2b ) and they are due to built-in stress in the ITO film. ( c ) Devices bent to 10 mm ( ε =0.25%). ( d ) Devices bent to 6 mm ( ε =0.4%). ( e ) Transfer characteristic ( V DS =0.1, 5 V) of a W/L =280 μm/60 μm transparent TFT, which is measured on Si, flat on polyimide after transfer and then bent to 10 and 6 mm (tensile strain parallel to the channel). Higher strain levels provoke cracks and delamination of the ITO. ( f ) Output characteristics for V GS =1, 1.5, 2 V of the device shown in e . ( g – i ) The transfer yield is about 50% (10 devices out of 20 work after transfer). The most remarkable changes, after the transfer, are observed in the increase of the gate leakage, I G , (( i ) plot in logarithmic scale) and of the off-current, I off , (( h ) plot in logarithmic scale). Threshold voltage, V TH , remains, instead, stable and average mobility, μ , is of about 16 cm 2 V −1 s −1 , which is lower than the Ti/Au metallization because of the increased contact resistance. Errors bars in the plots indicate the s.d. Full size image Highly flexible electronics After studying the maximum strain that both transparent and non-transparent devices can stand, we investigated the ultimate minimum bending radius if the bare parylene membrane is used as substrate. We expect a much higher flexibility for thinner substrates. In fact, our calculation (see Methods ) shows that for a 1μm thick parylene the 0.4% limit, registered for ITO transistors, is reached at a bending radius of about 50 μm [33] . In order to experimentally prove this finding, we transferred the membrane on top of a glass support where some fragments of human hairs had been placed. The membrane exhibits good conformability and it wraps around the hairs, which have a radius of about 50 μm ( Fig. 4a,b ). We repeated the experiment for non-transparent ( Fig. 4c ) and transparent TFTs ( Fig. 4e ). Both kinds of transistors, whose gate region is bent around the hairs, are fully operational. A transistor with Ti/Au contacts is reported in Fig. 4d . The device shows a mobility of 26 cm 2 V −1 s −1 and I on / I off ratio greater than 10 6 . A transparent device, instead, exhibits a mobility of 11 cm 2 V −1 s −1 and I on / I off greater than 10 4 ( Fig. 4f ). Interestingly, in both cases, the gate leakage current remains below 10 pA for the full range of operation proving that the gate dielectric properties are not degraded even after 10 voltage cycles (see Supplementary Fig. S4 ). These findings demonstrate that our technique enables the realization of high-performance TFTs, which withstand bending radii of 50 μm and can pave the way to ultra flexible and transparent displays. Furthermore, the thin substrate confers extreme conformability, which is particularly important for sensing in biological tissues. 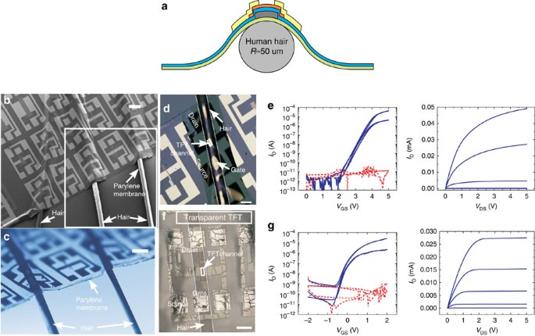Figure 4: Ultra flexible and transparent TFTs. (a) Schematic representation of a transistor wrapped round a human hair. (b) Scanning electron microscopy picture of transistors wrapped around three fragments of human hairs placed on a glass support. The thin membrane ensures high flexibility and conformability and it wraps around the hairs, which have a radius of ~50 μm (tensile strain,ε=0.4%) (scale bar, 200 μm). (c) Optical microscope picture of the area highlighted by the white box inb(scale bar, 200 μm). (d) Optical microscope picture of a non-transparent TFT (Ti/Au metallization) whose channel is bent around a hair (scale bar, 100 μm). (e) Transfer (VDS=0.1, 5 V) and output (VGS=3.5, 4, 4.5, 5 V) characteristics of a non-transparent TFT (W/L=280 μm/80 μm) bent around a hair. The device shows a threshold voltage,VTH, of about 3.4 V, a mobility,μ, of about 26 cm2V−1s−1, aIon/Ioffratio greater than 106and a gate leakage current,IG, smaller than 10 pA for full range of operations. The relatively high threshold voltage is due to the fact that this device is not passivated. (f) Transparent TFT whose channel region is bent around a hair (scale bar, 100 μm). (g) Transparent TFT (W/L=280 μm per 80 μm), when bent around a hair, shows a threshold voltage of 0.17 V and an effective mobility of 11 cm2V−1s−1. Figure 4: Ultra flexible and transparent TFTs. ( a ) Schematic representation of a transistor wrapped round a human hair. ( b ) Scanning electron microscopy picture of transistors wrapped around three fragments of human hairs placed on a glass support. The thin membrane ensures high flexibility and conformability and it wraps around the hairs, which have a radius of ~50 μm (tensile strain, ε =0.4%) (scale bar, 200 μm). ( c ) Optical microscope picture of the area highlighted by the white box in b (scale bar, 200 μm). ( d ) Optical microscope picture of a non-transparent TFT (Ti/Au metallization) whose channel is bent around a hair (scale bar, 100 μm). ( e ) Transfer ( V DS =0.1, 5 V) and output ( V GS =3.5, 4, 4.5, 5 V) characteristics of a non-transparent TFT ( W/L =280 μm/80 μm) bent around a hair. The device shows a threshold voltage, V TH , of about 3.4 V, a mobility, μ , of about 26 cm 2 V −1 s −1 , a I on / I off ratio greater than 10 6 and a gate leakage current, I G , smaller than 10 pA for full range of operations. The relatively high threshold voltage is due to the fact that this device is not passivated. ( f ) Transparent TFT whose channel region is bent around a hair (scale bar, 100 μm). ( g ) Transparent TFT ( W/L =280 μm per 80 μm), when bent around a hair, shows a threshold voltage of 0.17 V and an effective mobility of 11 cm 2 V −1 s −1 . Full size image The mechanical properties of the thin substrate are further investigated by transferring the devices onto a 100-μm thick polypropylene foil. This facilitates the handling and manipulation of the membrane while minimizing the strain induced by the substrate, thanks to the poor adhesion between polypropylene and parylene. The membrane on the polypropylene foil is folded to a radius of 750 μm ( Fig. 5a ), then repeatedly crumpled in the hands ( Fig. 5b ) and finally re-flatten ( Fig. 5c ). After the curling, we were able to measure only the non-transparent transistors while none of the transparent devices was functioning. We noticed cracks and delamination of the ITO layer after the experiment (see Supplementary Fig. S4 ), which could be caused by strain greater than the 0.4% limit. The transfer and output characteristics of a transistor with Ti/Au contacts are shown in Fig. 5e . The TFTs continue to function showing a quite stable threshold voltage and mobility ( Fig. 5f ) but with an increased gate leakage current ( Fig. 5g ). This could be explained by a partial deterioration of the gate dielectric that however, does not preclude the devices to continue working properly. After mechanical tests and measurements, the membrane can be smoothly released from the polypropylene substrate by dipping it in water and because of the poor adhesion ( Fig. 5d ). 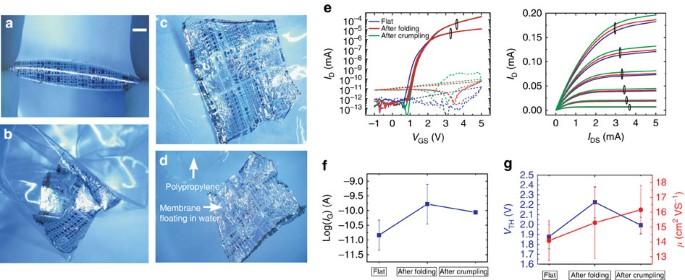Figure 5: Crumpling and curling the electronics. (a–d) The membrane is transferred on a 100-μm thick polypropylene foil, which is folded in hand (bending radius is about 750 μm), (scale bar, 1 mm). (b) The electronics is aggressively crumpled in hands. (c) Reflattening after crumpling. (d) The adhesion between the foil and the parylene surface is poor, hence, the strain arising from the substrate is reduced and the membrane can be released in water after the mechanical tests. The experiments are repeated for non-transparent and transparent devices but in the second case the aggressive crumpling provokes cracks and delamination of ITO layer (seeSupplementary Fig. S5). (e) Transfer (VD=0.1 V) and output characteristic (VGSfrom 3–5 with a 0.5 V step) of a non-transparent TFT. The device (W/L=50 μm/4 μm) continues to work after being folded and crumpled. (f,g) After crumpling, six devices out of 10 continue to work. Metal delamination and cracks in the active layers are the cause of failure. Gate leakage,IG, (logarithmic scale in the plot) increases more than one order of magnitude while threshold voltage,VTH, remains quite stable (±150 V in average). Average mobility,μ, is about 15 cm2V−1s−1and the change, after the mechanical test, remains in the range of ±2.5 cm2V−1s−1. Errors bars in the plots indicate the s.d. Figure 5: Crumpling and curling the electronics. ( a – d ) The membrane is transferred on a 100-μm thick polypropylene foil, which is folded in hand (bending radius is about 750 μm), (scale bar, 1 mm). ( b ) The electronics is aggressively crumpled in hands. ( c ) Reflattening after crumpling. ( d ) The adhesion between the foil and the parylene surface is poor, hence, the strain arising from the substrate is reduced and the membrane can be released in water after the mechanical tests. The experiments are repeated for non-transparent and transparent devices but in the second case the aggressive crumpling provokes cracks and delamination of ITO layer (see Supplementary Fig. S5 ). ( e ) Transfer ( V D =0.1 V) and output characteristic ( V GS from 3–5 with a 0.5 V step) of a non-transparent TFT. The device ( W/L =50 μm/4 μm) continues to work after being folded and crumpled. ( f , g ) After crumpling, six devices out of 10 continue to work. Metal delamination and cracks in the active layers are the cause of failure. Gate leakage, I G , (logarithmic scale in the plot) increases more than one order of magnitude while threshold voltage, V TH , remains quite stable (±150 V in average). Average mobility, μ , is about 15 cm 2 V −1 s −1 and the change, after the mechanical test, remains in the range of ±2.5 cm 2 V −1 s −1 . Errors bars in the plots indicate the s.d. Full size image The membrane is also light, and biocompatible [31] , [32] and can be transferred on arbitrary shaped, organic or inorganic tissues. To design a concrete application that takes advantages of such capabilities, we transferred the parylene membrane, with on top transparent transistors and strain gauge sensors, on a commercially available plastic contact lens ( Fig. 6 ). The membrane plus the devices have a total thickness of 1,145 nm. The strain gauge sensor consists of a Ti/Au (10 nm per 60 nm) stack and its response to applied strain ( Fig. 6c ) can be used to monitor the intraocular pressure. After transferring the lens onto an artificial eye ( Fig. 6b ), TFTs continue to function ( Fig. 6d,e ) and could be used for signal amplification in future developments. In the design of a real system, particular attention must be paid to the packaging, which has to mitigate or eliminate the effects of the aqueous humour of the eye (see Supplementary Fig. S7 ). Thereby, the developed technology could find application as smart contact lenses [36] able to monitor and diagnose glaucoma disease and it could offer significant advantages over existing solutions ( http://www.sensimed.ch ) in terms of thickness, lightness and transparency and, hence, comfort for the patient. 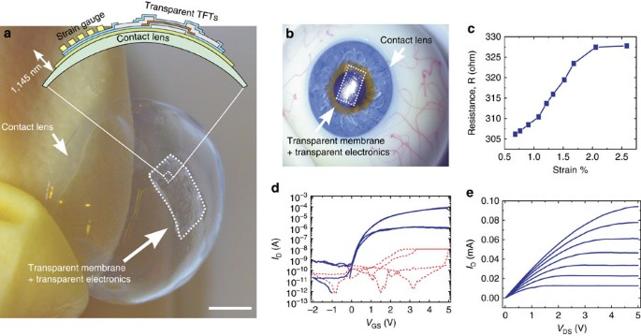Figure 6: Transparent and light electronics for smart contact lens. (a) The membrane with on top transparent TFTs and gold strain gauge sensors is transferred on a plastic contact lens held between two fingers (scale bar, 2.5 mm). (b) The membrane transferred on an artificial eye. (c) Strain gauge sensor response to applied strain. The sensor can be potentially exploited to monitor the intraocular pressure. (d,e) Transparent TFT (W/L=280 μm/80 μm) measured on a contact lens placed on an artificial eye. The transfer characteristic refers toVDS=0.1 and 5 V while the output characteristic is forVGSfrom 2–5 V with a 0.5 V step. The transistor exhibits a mobility of about 7.2 cm2V−1s−1, a threshold voltage of 0.34 V, a sub-threshold swing of 172 mV/dec, an on/off ratio greater than 105and a transconductance of about 0.15 μS/μm atVGS=5 V. Figure 6: Transparent and light electronics for smart contact lens. ( a ) The membrane with on top transparent TFTs and gold strain gauge sensors is transferred on a plastic contact lens held between two fingers (scale bar, 2.5 mm). ( b ) The membrane transferred on an artificial eye. ( c ) Strain gauge sensor response to applied strain. The sensor can be potentially exploited to monitor the intraocular pressure. ( d , e ) Transparent TFT ( W/L =280 μm/80 μm) measured on a contact lens placed on an artificial eye. The transfer characteristic refers to V DS =0.1 and 5 V while the output characteristic is for V GS from 2–5 V with a 0.5 V step. The transistor exhibits a mobility of about 7.2 cm 2 V −1 s −1 , a threshold voltage of 0.34 V, a sub-threshold swing of 172 mV/dec, an on/off ratio greater than 10 5 and a transconductance of about 0.15 μS/μm at V GS =5 V. Full size image In conclusion, we proposed a wafer-scale methodology to fabricate electronics on an engineered substrate, which is designed to enable the release, the transfer and the adhesion of electronics onto biological tissues, plastic foils and any shaped rigid or flexible objects. Thanks to this approach, we were able to fabricate high-performance devices and circuits on a 1-μm thick parylene film. Such electronics simultaneously exhibit unique capabilities as ultra-flexibility, transparency, conformability, lightness and biocompatibility. Transparent transistors and strain gauge sensors were transferred on plastic contact lenses, which could potentially serve to monitor the intraocular pressure and detect and diagnose glaucoma disease. The smart contact lens application, demonstrated here, presents just one example of the type of system that can be realized by the reported process scheme. Ultralight solar cells, implantable devices, smart-skin and electronic textiles are also envisioned as possible future applications. Device fabrication The carrier chip, used during the experiments, is a 2-inch silicon wafer. The PVA (12% concentration in water) and PVAc (4% concentration in methanol) are spin coated at 4,000 r.p.m. for 60 s and subsequently baked at 100 °C for 120 s. Parylene is thermally evaporated. PVAc is only used in case of transfer onto polyimide foil and nitride rubber, skin and plant leaves. After use, it can be safely removed by diluted acetic acid. Thin film transistor consists of a 35 nm Cr bottom gate deposited by e-beam evaporation; Al 2 O 3 (thickness: 25 nm, dielectric constant: 9.5) is used as gate oxide and deposited at 150 °C, which is the highest temperature encountered during the fabrication. Contact Vias: Opennings through the oxide to get access to the contact pads by a 50 ml H 2 O+45 ml CH 3 COOH (acetic acid)+10 ml HNO 3 (nitric acid)+250 ml H 3 PO 4 (phosphoric acid) solution, heated to a temperature of 50 °C. Amorphous-IGZO (15 nm) is RF magnetron sputtered at room temperature and without any subsequent annealing step, patterned and etched by a HCl:DI water (1:120) solution. Source and drain contacts consist of Ti/Au 10 nm/60 nm metal layers structured by acetone lift-off. For the layer structuring, standard UV lithography is used. In transparent TFTs, the metal for gate, source and drain are replaced by ambient temperature-sputtered indium tin oxide (100 nm). Transfer technique In order to facilitate the PVA dissolution the wafer is mechanically scratched at the border. Once PVA is dissolved and the membrane released, the transfer is done by moving the destination substrate or support beneath the flexible electronic membrane and then by lifting the flexible electronic membrane out of the water. The membrane can be consecutively transferred from one substrate to another till it dries completely. The transfer of the membrane onto the polyimide and the polypropylene foils is followed by a baking step at 70 °C for 10 min. Electrical characterization The device characterization is performed with an Agilent Semiconductor Analyser and with gold probe tips. The differential amplifier is measured with two active probes ( C ⩽ 2 pF, R =1 MΩ). Strain level calculation For the calculation of the strain level in TFTs, we used a simplified version of the formula contained in the work of Gleskova et al . [33] : where the term χ and γ are defined as χ = Y f / Y s and γ = d f / d s . R is the bending radius, d f and d s are the thickness of TFT and of the substrate, respectively, Y f and Y s are the Young’s modulus of TFT layers (weighted average of all deposited materials) and of the substrate, respectively. We used Y s =400 kPa for parylene and Y s =2.5 Gpa for polyimide. Mechanical bending All the devices are bent in such a way that the strain is tensile and parallel to the channel of the TFTs. No experiments have been performed in case of perpendicular strain. Circuits are designed in such a way all the TFTs are aligned in the same direction. The mechanical stability range for non-transparent devices is 0.5% tensile strain parallel to the TFT channel and for transparent TFTs the limit is 0.4%. Curling experiment is more qualitative than quantitative and no exact estimation of the modulus and direction of the strain is possible. Failure mechanisms, in case of ITO based devices, can be strain, which is greater than 0.4% or a perpendicular component, which is responsible of cracks, which disconnect the source from the drain. How to cite this article : Salvatore, G. A. et al . Wafer-scale design of lightweight and transparent electronics which wraps around hairs. Nat. Commun. 5:2982 doi: 10.1038/ncomms3982 (2014).